Dynamic self-stiffening in liquid crystal elastomers Biological tissues have the remarkable ability to remodel and repair in response to disease, injury and mechanical stresses. Synthetic materials lack the complexity of biological tissues, and man-made materials that respond to external stresses through a permanent increase in stiffness are uncommon. Here we report that polydomain nematic liquid crystal elastomers increase in stiffness by up to 90% when subjected to a low-amplitude (5%), repetitive (dynamic) compression. Elastomer stiffening is influenced by liquid crystal content, the presence of a nematic liquid crystal phase and the use of a dynamic as opposed to static deformation. Through rheological and X-ray diffraction measurements, stiffening can be attributed to a mobile nematic director, which rotates in response to dynamic compression. Stiffening under dynamic compression has not been previously observed in liquid crystal elastomers and may be useful for the development of self-healing materials or for the development of biocompatible, adaptive materials for tissue replacement. Biological tissues have the remarkable ability to remodel and repair in response to disease, injury and mechanical stresses [1] , [2] , [3] . Well-known examples include bone remodelling and strengthening through a process that involves changes in bone mass and porosity [4] , and muscle development, tumour growth and blood vessel structure are all affected by mechanical stresses [5] , [6] , [7] . Synthetic materials lack the complexity of biological tissues, and man-made materials that respond to external stresses through a permanent increase in stiffness are uncommon [8] , [9] . Here, we report that polydomain nematic liquid crystal elastomers (LCEs) increase in stiffness by up to 90% when subjected to a low-amplitude (5%), repetitive (dynamic) compression. Such self-stiffening is uncharacteristic of synthetic rubbers [9] , [10] but arises in polydomain LCEs due to the presence of a mobile nematic director that re-orients in response to external stresses. The observed dynamic stiffening in polysiloxane LCEs may be useful for the development of self-healing materials and biocompatible, adaptive materials for tissue replacement. Additionally, the use of low strain, repetitive compression represents a facile method to prepare uniformly aligned LCEs, which are typically prepared by applying large tensile strains or external fields during material synthesis [11] , [12] , [13] , [14] , [15] , [16] . Previous work has focused on the properties of LCEs under large-strain deformation, but our findings indicate rich behaviour at previously overlooked low strain, dynamic deformations. LCEs are comprised of a crosslinked network of flexible polymer chains with liquid crystalline order ( Fig. 1a ) [17] , [18] . Polydomain LCEs were prepared by coupling liquid crystal mesogens to poly(hydrogenmethylsiloxane) (PHMS) ( Fig. 1a ), as has been previously reported [19] . The resulting materials are rubbery ( T g ≈−30 °C), nematic networks with no global orientation of the nematic director (polydomain). Nematic order fundamentally alters the response of LCEs to external stresses. Network chains in LCEs are locally anisotropic and assume an ellipsoidal conformation, in contrast to the spherical random coil conformation of conventional isotropic rubbers. LCEs exhibit ‘soft elasticity’ that is exemplified by large-strain deformations with little resistance [17] , [20] , [21] . Herein, we examine the behaviour of polydomain LCEs under a repetitive, compressive deformation at low strains (5%). We find a significant increase in stiffness after extended compression and, through a combination of dynamic mechanical testing (DMA), two-dimensional wide-angle X-ray diffraction (2DWAXD) and polarized optical microscopy, can attribute microstructure changes to a mobile nematic director, which re-orients in response to dynamic stresses. 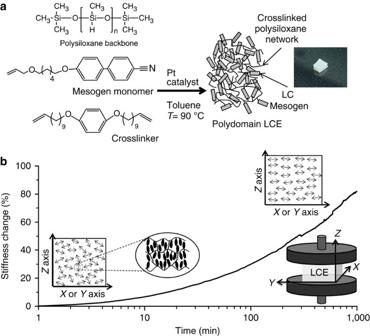Figure 1: Synthesis and dynamic strain stiffening of polydomain LCEs. (a) Schematic for the synthesis of a polydomain LCE. A representative LCE sample is shown on the right-hand side, and DMA was carried out on LCEs with dimensions of 1.5 × 1.5 × 1 mm3. (b) Change in stiffness (%) versus time for a LCE (LCE90) under repetitive (dynamic) compression. The LCE is dynamically compressed between two flat plates at 5 Hz, 45 °C, a preload of 0.01 N, and a 5% strain amplitude using a DMA Q800. Schematics in the bottom-left and top-right show the alignment of nematic domains in LCEs subjected to repetitive compression. The inset in the bottom right shows schematic of experimental protocol employed for the dynamic compression of polydomain LCEs. The data shown are plotted on linear-log axes, and data on linear-linear axes are provided in theSupplementary Fig. S5. A plot of the time-dependent strain applied to the sample during measurement is shown inSupplementary Fig. S6. Figure 1: Synthesis and dynamic strain stiffening of polydomain LCEs. ( a ) Schematic for the synthesis of a polydomain LCE. A representative LCE sample is shown on the right-hand side, and DMA was carried out on LCEs with dimensions of 1.5 × 1.5 × 1 mm 3 . ( b ) Change in stiffness (%) versus time for a LCE (LCE90) under repetitive (dynamic) compression. The LCE is dynamically compressed between two flat plates at 5 Hz, 45 °C, a preload of 0.01 N, and a 5% strain amplitude using a DMA Q800. Schematics in the bottom-left and top-right show the alignment of nematic domains in LCEs subjected to repetitive compression. The inset in the bottom right shows schematic of experimental protocol employed for the dynamic compression of polydomain LCEs. The data shown are plotted on linear-log axes, and data on linear-linear axes are provided in the Supplementary Fig. S5 . A plot of the time-dependent strain applied to the sample during measurement is shown in Supplementary Fig. S6 . Full size image Dynamic stiffening of polydomain LCEs To investigate the role of mesogen content on mechanical properties, a systematic series of polydomain LCEs (LCE90, LCE80, LCE60, LCE40 and LCE20) were prepared with mesogen content ranging from 90 to 20 mol % relative to the Si–H bonds in the PHMS polymer ( Table 1 ). Poly(dimethyl siloxane) (PDMS) was also studied for comparison with the LCEs. PDMS is chemically and mechanically similar to the LCEs studied, but with no mesogen content. Under 16 h of repetitive, compressive loading (5 Hz, 5% strain), LCE90 exhibits a 90% increase in stiffness ( Fig. 1b ). The strain amplitude is maintained at 5% for the duration of the experiment. As shown in Table 1 , the final stiffness of LCE90 surpasses the initial values of other LCEs studied despite the lower crosslink density of LCE90. DMA of all LCEs prepared shows that mesogen content is correlated with increased stiffness, in particular for the series of samples where the crosslink density is held constant (LCE20, LCE40 and LCE60) ( Fig. 2 ). LCE60 and LCE80 exhibit a similar, although less pronounced, stiffening response compared with LCE90. The stiffness increase under 5% compressive loading is 63% and 33% for LCE80 and LCE60, respectively. LCE20 and LCE40, both with no nematic phase ( Supplementary Fig. S1 ), exhibit a stiffness increase of only 14%. Finally, PDMS exhibits a stiffness increase of only 1.4%. Table 1 Characteristics of LCEs and PDMS. 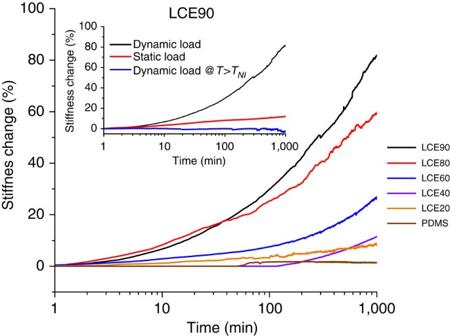Figure 2: Dynamic strain stiffening in LCEs with varying mesogen content. Change in stiffness (%) versus time for a series of LCEs varying in mesogen content and PDMS under dynamic compressive strain. The data shown are plotted on linear-log axes, and data on linear-linear axes are provided in theSupplementary Fig. S4. The extent of stiffening is correlated with LCE mesogen content. Measurements were carried out at 5 Hz, 45 °C and at 5% strain amplitude. The top inset compares dynamic strain stiffening in LCE90 under dynamic load, static load and dynamic load aboveTNI(80 °C) and demonstrates that stiffening is only observed in the nematic phase under dynamic compression. For static load tests, samples were subjected to a compressive strain of 6%, both greater than the corresponding stress and strain values applied during dynamic loading. Full size table Figure 2: Dynamic strain stiffening in LCEs with varying mesogen content. Change in stiffness (%) versus time for a series of LCEs varying in mesogen content and PDMS under dynamic compressive strain. The data shown are plotted on linear-log axes, and data on linear-linear axes are provided in the Supplementary Fig. S4 . The extent of stiffening is correlated with LCE mesogen content. Measurements were carried out at 5 Hz, 45 °C and at 5% strain amplitude. The top inset compares dynamic strain stiffening in LCE90 under dynamic load, static load and dynamic load above T NI (80 °C) and demonstrates that stiffening is only observed in the nematic phase under dynamic compression. For static load tests, samples were subjected to a compressive strain of 6%, both greater than the corresponding stress and strain values applied during dynamic loading. Full size image The presence of nematic order and the application of a repetitive (dynamic) load are essential to the stiffening response ( Fig. 2 ). As shown in Fig. 2 (inset), LCE90 exhibits a modest increase in stiffness when dynamically compressed in the isotropic phase at 80 °C (~15%, similar to LCE20 and LCE40) while stiffness increases by >80% when the same measurement is carried out in the nematic phase at 45 °C. This same trend is observed for all nematic LCEs (see Supplementary Fig. S2 ). Furthermore, stiffening is only observed under dynamic, compressive stress. An extended static compression test with an applied stress greater than the maximum stress applied during dynamic compression (70 kPa) and a strain of 6% resulted in only a modest (~10%) stiffness increase (see inset of Fig. 2 and Supplementary Fig. S2 ). Thus, consistent with previous reports [14] , [15] , a static deformation at low strain (<10%) does not result in significant changes to the microstructure of the LCE. As an additional control experiment, samples held at 45 °C for at least 16 h in the DMA without compression show no stiffness increase. LCE microstructure analysis Microstructure changes in polydomain LCEs were analysed by 2DWAXD before and after deformation. In the experimental configuration used for this study, scattering peaks corresponding to mesogen spacing along the molecular width are clearly resolved ( Fig. 3 ), enabling quantification of orientational ordering of the mesogenic side-groups. X-ray scattering measurements were performed using a Rigaku Raxis-IV++ equipped with an incident beam monochromator, pinhole collimation (0.3 mm) and Cu X-ray tube ( λ =1.54 Å). The sample to detector distance was 100 mm. Before compressive deformation, all LCEs exhibit an isotropic scattering peak characteristic of a polydomain, nematic LCE ( Fig. 3a ). After dynamic compression, a clear anisotropy emerges in LCE90, LCE80 and LCE60 (see Fig. 3c ). Anisotropic scattering is only observed in the x – z and y – z planes, but the scattering pattern in the x – y plane remains isotropic. This indicates that the nematic director in these samples rotates away from the z axis (compressive direction) to lie primarily in the x – y plane but remains globally disordered in the x – y plane, resulting in an oblate LC orientation after dynamic compression. The reorientation of the LC side-groups can also be followed qualitatively through polarized optical microscopy; global reorientation of the nematic director away from the z axis is consistent with reduced light transmission through the x – z and y–z faces when crossed polarizers are aligned with the axis of compression ( Fig. 3b ). 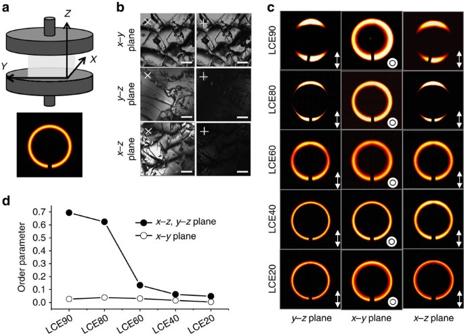Figure 3: Microstructure analysis of LCEs after dynamic compression. (a) Schematic of geometry during dynamic compression experiment and 2DWAXD pattern of unstressed, polydomain LCE90. All LCEs exhibit similar 2DWAXD patterns before dynamic compression. (b) Polarizing optical microscopy images of dynamically stressed LCE90 along three different faces. Reduced light transmission through thex–zandy–zfaces when crossed polarizers are oriented parallel to the compression direction (zaxis) indicates reorientation of the nematic director perpendicular to thezaxis. All scale bar, 0.1 mm. (c) 2DWAXD patterns of LCEs with varying mesogenic content subjected to compressive dynamic load (5 Hz, 5% strain) for at least 16 h. The patterns are shown for three independent LCE faces (x–zplane,x–yplane andy–zplane), and the arrow on the bottom right-hand side indicates the direction of compression. The anisotropic scattering pattern observed for thex–zandy–zplanes indicates that the LCE nematic director rotates away from thezaxis (compressive direction) to lie primarily in thex–yplane, but the nematic director remains disordered in thex–yplane. (d) Macroscopic alignment parameterSfor dynamically stressed LCEs extracted from model fit of 2DWAXD pattern. The order parameterSis defined with respect to thex–yplane. The order parameters for thex–zandy–zplanes is an average of the order parameters measured in each plane. Figure 3: Microstructure analysis of LCEs after dynamic compression. ( a ) Schematic of geometry during dynamic compression experiment and 2DWAXD pattern of unstressed, polydomain LCE90. All LCEs exhibit similar 2DWAXD patterns before dynamic compression. ( b ) Polarizing optical microscopy images of dynamically stressed LCE90 along three different faces. Reduced light transmission through the x – z and y–z faces when crossed polarizers are oriented parallel to the compression direction ( z axis) indicates reorientation of the nematic director perpendicular to the z axis. All scale bar, 0.1 mm. ( c ) 2DWAXD patterns of LCEs with varying mesogenic content subjected to compressive dynamic load (5 Hz, 5% strain) for at least 16 h. The patterns are shown for three independent LCE faces ( x – z plane, x–y plane and y–z plane), and the arrow on the bottom right-hand side indicates the direction of compression. The anisotropic scattering pattern observed for the x – z and y – z planes indicates that the LCE nematic director rotates away from the z axis (compressive direction) to lie primarily in the x – y plane, but the nematic director remains disordered in the x–y plane. ( d ) Macroscopic alignment parameter S for dynamically stressed LCEs extracted from model fit of 2DWAXD pattern. The order parameter S is defined with respect to the x – y plane. The order parameters for the x – z and y – z planes is an average of the order parameters measured in each plane. Full size image Coupling between elastomer deformation and nematic director orientation The dynamic mechanical analysis measurements together with WAXD patterns for stressed and unstressed LCEs establish a clear connection between stiffening and reorientation of the nematic LC director. In LCEs, network chain conformation is coupled to the nematic director orientation. Therefore, the observed reorientation of the mesogenic side-groups perpendicular to the compressive axis reflects a reorientation of the LCE network chains ( Fig. 4c ). The strain lines corresponding to a linear, compressive deformation can be calculated by performing finite element modelling simulations using COMSOL Multiphysics 4.2 simulation package. Simulation results predict elongational strains in the plane perpendicular to the compressive axis. This elongational strain is expected to preferentially align the ellipsoidal LCE network chains in the x – y plane and, due to coupling between the LC side-group and polymer backbone, result in the observed reorientation of the nematic director. 2DWAXD images indicate reorientation of the LC side-groups in the x – y plane, consistent with a preferential orientation of the LC side-groups parallel to the polymer backbone. The 2DWAXD data also enable calculation of a macroscopic alignment parameter , averaged over the entire sample, where θ is the angle between the local director orientation and the x – y plane [22] , [23] . The increase in macroscopic alignment is directly correlated with mesogen content, as shown in Fig. 3d . Furthermore, the coupling between mesogen side-group orientation and polymer orientation results in macroscopic changes to sample dimensions. As shown in the Supplementary Table S1 , dimensional changes up to 8.3% along compression (measure along z axis) and 7.7% along x and y axes are recorded, consistent with the coupling of macroscopic shape and global director orientation. As the stiffening response arises due to a director reorientation, stiffening is fully reversible. This is demonstrated by the observed relaxation of a sample subjected to dynamic compression: after 3 months, the stiffness returns to its initial value and the director orientation is polydomain ( Supplementary Fig. S3 ). 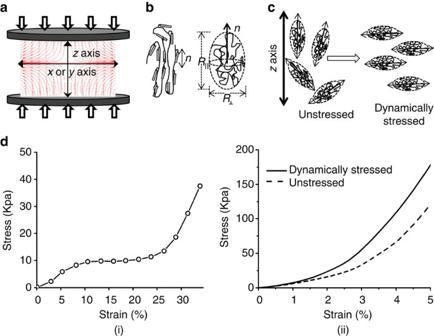Figure 4: Reorientation of LC polymer chains under dynamic compression. (a) Finite element modeling (FEM) simulation showing stress lines as a result of compression. FEM simulations were performed out using COMSOL Multiphysics 4.2 simulation package. (b) Schematic depiction of a prolate LC polymer chain. Note that the mesogenic side-groups are oriented preferentially parallel to the polymer backbone. (c) Reorientation of prolate LC polymer chains under compressive strain. (d) Stress–Strain relationship of (i) polydomain LCE under uniaxial tension (data reproduced with permission from Clarkeet al.29) and (ii) polydomain LCE90 before and after dynamic compression. For LCE90 stress–strain profiles are recorded along the compression axis. Similar relaxation is observed for a dynamically stressed sample annealed above the T NI for 4 h. Figure 4: Reorientation of LC polymer chains under dynamic compression. ( a ) Finite element modeling (FEM) simulation showing stress lines as a result of compression. FEM simulations were performed out using COMSOL Multiphysics 4.2 simulation package. ( b ) Schematic depiction of a prolate LC polymer chain. Note that the mesogenic side-groups are oriented preferentially parallel to the polymer backbone. ( c ) Reorientation of prolate LC polymer chains under compressive strain. ( d ) Stress–Strain relationship of (i) polydomain LCE under uniaxial tension (data reproduced with permission from Clarke et al . [29] ) and (ii) polydomain LCE90 before and after dynamic compression. For LCE90 stress–strain profiles are recorded along the compression axis. Full size image The stiffening response can be understood within the theoretical framework of nematic rubber elasticity [17] . Warner et al . [17] showed that for nematic LCEs, the free energy density satisfies the following equation: , where μ is the rubber elastic modulus, λ is strain and is the network step-length tensor that describes the local (generally anisotropic) chain conformation. This theory assumes Gaussian, phantom network chains and the absence of quenched disorder. A consequence of this free energy expression is that strains λ of the form , where W α is an arbitrary rotation by an angle α , come with no increase to the elastic free energy. Thus, for this type of strain, the LCE deforms ‘softly’ with no resistance. This result only applies to the ideal case, but real elastomers more commonly exhibit semi-soft elasticity, with some resistance to deformation below a threshold stress value. An example of this for a polydomain LCE under uniaxial strain is shown in Fig. 4d ; the elastomer exhibits, after a strain threshold, a pronounced plateau in the stress. This stress plateau is a direct result of ‘soft elasticity’ and is associated with nematic director rotations. At higher strains, the nematic director is fully aligned, and director reorientations can no longer accommodate further strain, resulting in a stress increase. This particular example reflects the behaviour of LCEs under large (>10%) uniaxial strains but similar behaviour is observed in the present study for LCEs under compression. In initially unstressed samples, a ‘soft’ elastic response is observed. The softness or reduced stiffness is a result of a globally disordered nematic director that can accommodate deformations through rotation. However, extended dynamic compression results in a reorientation of the nematic director and a corresponding increase in stiffness ( Fig. 4d ). Similar to the behaviour of LCEs under uniaxial tension, reorientation of the nematic director is associated with an increased resistance to deformation. A comparison of deformed and undeformed LCEs shows that the measured stiffness increase is a distinctly nonlinear phenomenon. As shown in Fig. 4d and the Supplementary Fig. S3 , there is no difference in stiffness between stressed and unstressed samples for strain values <1%. Thus, as expected, at low compressive strains LCEs behave linearly, and the slope of the stress–strain curve simply reflects the equilibrium Young’s modulus. Differences between stressed and unstressed LCEs are only observed for strain values greater than ~2%. This threshold value may reflect ’semi-softness‘ in LCEs, which arises due to polymer chain length polydispersities, compositional fluctuations and other network non-idealities. Strain stiffening in LCEs contrasts with the irreversible softening of polymeric networks under cyclic strain, a phenomenon known as the Mullins effect [9] , [10] , [24] . Although the Mullins effect is not fully understood [9] , [10] , it has been seen in crystallizable rubbers or rubbers with added fillers and has also been observed in biological tissue [25] , [26] . Recently, stiffening behaviour was reported for bundled actin networks under cyclic shear [27] . This was observed at higher crosslink densities and attributed to the physical nature of the network, which allowed reorganiation of the network constituents, resulting in hardening after cyclic shear [27] . This contrasts with the dynamic stiffening reported here in covalent LCE networks. The novelty of the present work is the discovery of dynamic stiffening in a synthetic, homogeneous polymeric network with liquid crystalline order. Additionally, the presence of liquid crystal order enables quantitative characterization of side-group and network chain orientation before and after deformation, establishing a direct connection between stiffening and network chain conformation. In summary, we report LCE self-stiffening in response to dynamic, compressive loading. The stiffening behaviour observed here is for a permanent network at low strains and can be attributed to a mobile nematic director. Director reorientation and alignment at low strains and dynamic compression has not been previously reported in LCEs and suggest underlying network relaxation modes at 5 Hz, which govern the response. LCEs that increase in stiffness may be useful for the development of self-healing materials or for the development of biocompatible, adaptive materials for tissue replacement. Dynamic compression is a straightforward method for preparing uniformly aligned nematic LCEs, and may be aplicable to higher-order liquid crystal phases, including chiral nematics and smectics. Other repetitive deformations (for example, uniaxial tension, shear) at low strain values may lead to similar director reorientations in LCEs and will be the focus of future work. Materials Toluene, Pt-catalyst ((dichloro (1, 5-cyclooctadiene) platinum (II)), allylbromide, butanol, 11-bromo-1-undecene, sodium hydride (60% dispersion in mineral oil), hydroquinone, magnesium sulphate, PHMS (poly (hydromethylsiloxane)) ( M w =1,700–3,200 g per mole), ethyl acetate, 4-hydroxyl-4′-cyano biphenyl, sodium hydroxide, tetrahydrofuran, diethyl ether, dimethyl formamide (DMF), 6-bromo-1- hexanol, benzene, methanol and potassium carbonate were purchased from commercial suppliers and used as received. The crosslinker (1,4-di(10-undecenyloxy)benzene) was synthesized as described previously [28] . 4-(1-Hexanol oxy)-4′-cyano biphenyl and mesogenic side-group were prepared as described below (see Supplementary Fig. S4 for reaction scheme). Preparation of 4-(1-hexanol oxy)-4′-cyano biphenyl (3) 4-Hydroxyl-4′-cyano biphenyl (1, 7 mmol, 1.36 g), 6-bromo-1-hexanol (2, 10 mmol, 1.83 g), and K 2 CO 3 (14 mmol, 1.934 g) were dissolved in 25 ml DMF and heated to 90 °C for 20 h. The reaction was then quenched by adding water and filtering to collect a white precipitate. The precipitate was then dried under vacuum and recrystallized in benzene to obtain the desired product. 1 H NMR (400 MHz, CDCl 3 ), δ (p.p.m. ): 7.8–7.6 (m, 4H) 7.54–7.50 (d, 2H), 7.0–6.9 (d, 2H), 4.20 (t, 2H), 3.36 (t, 2H), 1.8 (m, 2H), 1.7 (m, 2H), 1.40 (m, 4H). Preparation of mesogenic side-group (4) 3 (6 mmol, 1.77 g) was slowly added to a solution of sodium hydride (12.5 mmol, 0.3 g) in 30 ml diethyl ether/DMF (10:1). The reaction mixture was stirred under nitrogen atmosphere for 1 h before cooling to 0 °C and adding a solution of allylbromide (1.2 g, 10 mmol) in 5 ml diethyl ether dropwise. The reaction was allowed to proceed overnight before adding brine to quench the reaction. The layers were separated and the organic layer was washed with 1 N HCl and water. The product was concentrated under reduced pressure and purified by column chromatography (silica gel, eluent: ethyl acetate/hexanes 1:9 v/v). 1 H NMR (400 MHz, CDCl3), δ (p.p.m. ): 7.7-7.5 (m, 6H), 7.0–7.1 (d, 2H), 5.8 (m, 1H), 5.0 (d, 2H), 4.2 (t, 2H), 4.0 (d, 2H), 3.4 (t, 2H), 1.8–1.4 (m, 8H). Preparation of polydomain LCE Polydomain LCE samples were synthesized in the isotropic phase as described previously [19] . Briefly, mesogenic side-group ( 4 ), 4-(1-hexanol oxy)-4′-cyano biphenyl crosslinker and PHMS (poly (hydromethylsiloxane)) were dissolved in toluene along with the Pt-catalyst, and the reaction was allowed to proceed for 70 °C for 3 days. Elastomers were then swollen in dichloromethane for several days to wash out the unreacted materials and nonreactive solvent. By gradually increasing the methanol content of swelling solvent, elastomers were deswollen and then air-dried before testing. Dynamic mechanical analysis For the DMA studies, the samples were razor cut to dimensions of 1.5 × 1.5 × 1 mm 3 . All sample dimensions were measured using DMA and verified with a digital caliper. DMA was carried out in compression mode as illustrated in Fig. 1b using TA Instruments Q800 DMA at a 5% strain amplitude, 5 Hz requency and at a preload of 0.01 N. All the tests were conducted isothermally at 45 °C, except where otherwise noted. How to cite this article: Agrawal, A. et al . Dynamic self-stiffening in liquid crystal elastomers. Nat. Commun. 4:1739 doi: 10.1038/ncomms2772 (2013).